A nine-atom rhodium–aluminum oxide cluster oxidizes five carbon monoxide molecules Noble metals can promote the direct participation of lattice oxygen of very stable oxide materials such as aluminum oxide, to oxidize reactant molecules, while the fundamental mechanism of noble metal catalysis is elusive. Here we report that a single atom of rhodium, a powerful noble metal catalyst, can promote the transfer of five oxygen atoms to oxidize carbon monoxide from a nine-atom rhodium–aluminum oxide cluster. This is a sharp improvement in the field of cluster science where the transfer of at most two oxygen atoms from a doped cluster is more commonly observed. Rhodium functions not only as the preferred trapping site to anchor and oxidize carbon monoxide by the oxygen atoms in direct connection with rhodium but also the primarily oxidative centre to accumulate the large amounts of electrons and the polarity of rhodium is ultimately transformed from positive to negative. Oxide-supported rhodium (Rh) exhibits extraordinary catalytic activity in a large number of reactions [1] , [2] , [3] , [4] , [5] , [6] , [7] , [8] , [9] such as the oxidation of carbon monoxide (CO) [1] , [2] , [3] , [7] , carbon dioxide methanation [6] , partial oxidation of methane to syngas [4] , [5] , [8] , [9] and so on. It has been reported that trace amounts of Rh can promote direct participation of lattice oxygen of chemically very inert supports such as aluminum oxide (Al 2 O 3 ), to oxidize reactant molecules [4] , [5] , [9] , while the fundamental mechanism is elusive. Exploring the function of Rh in invoking the lattice oxygen of oxide support is of great importance to understand heterogeneous catalysis but remains a big challenge because of the structure complexity of bulk material. Atomic clusters are considered as the intermediate matter to bridge atoms and their bulk counterpart [10] , and can be ideal models for active sites of condensed-phase system. Cluster reactions [11] , [12] , [13] , [14] , [15] , [16] , [17] can be studied under isolated conditions to provide the mechanistic insights of elementary steps in the related condensed-phase systems. Important findings such as spin conservation [13] and the complementary active sites [15] have been revealed by studying the reactions of aluminum clusters with molecular O 2 and water, respectively. The oxygen atom transfer (OAT) from metal oxide clusters to small molecules is one type of extensively studied reactions [12] , [18] , [19] . Noble metal-doped heteronuclear oxide clusters [20] are being actively studied to understand the mechanistic nature of supported catalysts in the OAT reactions such as CO oxidation, an important model reaction in heterogeneous processes [21] and its wide applications in air purification. Au and Pt atoms have been emphasized to be crucial, to promote significantly the efficiency of OAT in CO oxidation [22] , [23] , [24] , [25] , [26] . However, each of the reported Au or Pt-doped clusters such as AuAl 3 O 5 + and PtAl 3 O 7 − can transfer at most two oxygen atoms to oxidize CO (refs 22 , 23 , 24 , 25 , 26 ). Here we report that a single Rh atom can unexpectedly promote the transfer of five oxygen atoms to oxidize CO from a nine-atom cluster RhAl 2 O 6 + , which produces the oxygen very deficient species RhAl 2 O + . In contrast, reported homonuclear aluminum oxide clusters (Al x O y ± ) [26] , [27] can deliver only one oxygen atom to CO and these reactive clusters such as Al 2 O 3 + and Al 4 O 7 − are all oxygen-rich species. Identification of multiple OAT from a single Rh-atom-doped cluster to reactant molecules is an important step to understand the participation of lattice oxygen promoted by noble metals. This gas-phase study that a nine-atom rhodium–aluminum oxide cluster oxidizes five CO molecules is a sharp improvement in the field of cluster science and provides a strictly molecular level understanding of the fundamental mechanism of noble metal catalysis in the related condensed phase. Reactivity of rhodium–aluminum oxide clusters with CO The RhAl 2 O m + ( m =2–6) cluster ions were generated by laser ablation of a mixed-metal disk compressed with Rh and Al powders. The generated RhAl 2 O m + cluster ions were mass-selected, cooled and then interacted with N 2 and CO in an ion trap reactor, as shown in Figs 1 and 2 . On the interaction of RhAl 2 O 6 + with 150 mPa N 2 ( Fig. 1a ), weak N 2 adsorption (RhAl 2 O 6 N 2 + ) and N 2 /O 2 exchange (RhAl 2 O 4 N 2 + ) products were generated. Generation of RhAl 2 O 4 N 2 + suggests the possible presence of superoxide (O 2 −· ) or peroxide (O 2 2− ) unit in RhAl 2 O 6 + (RhAl 2 O 6 + + N 2 → RhAl 2 O 4 N 2 + + O 2 ). In sharp contrast, on the interaction of RhAl 2 O 6 + with CO ( Fig. 1b–d ), a series of products, from RhAl 2 O 5 + to RhAl 2 O + , were generated gradually with the increase of CO partial pressure from 2 to 13 mPa. Signals RhAl 2 O 1–5 + did not appear on the interaction of RhAl 2 O 6 + with even high pressure N 2 ( Fig. 1a ). Additional experimental techniques such as multiphoton ionization [28] , [29] employing pulsed lasers are required to observe the neutral CO 2 molecules. However, N 2 experiment in Fig. 1a also indicates that products RhAl 2 O 1–5 + are due to the chemical reactions of RhAl 2 O 6 + with CO rather than collision-induced dissociation and RhAl 2 O 6 + may oxidize five CO molecules consecutively (equation (1)). 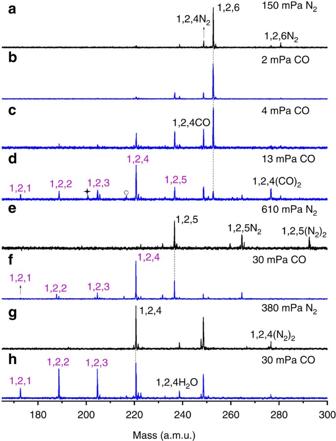Figure 1: Reactivity of RhAl2O4–6+clusters with CO. Time-of-flight mass spectra for reactions of mass selected RhAl2O4–6+with N2(a,e,g) and CO (b–d,f,h) are shown. Peaks marked with asterisk and hollow circle indare CO adsorption products of RhAl2OCO+and RhAl2O2CO+, respectively. RhxAlyOz+and RhxAlyOzX+(X=N2, CO and H2O) species are labeled asx,y,zandx,y,zX, respectively. Signal 1,2,4H2O inhis due to the residual water in the gas handling system. The time periods for reactions RhAl2O6++ CO, RhAl2O5++ CO and RhAl2O4++ CO were about 1.1, 0.7 and 0.6 ms, respectively. The reactant gas pressures are shown in mPa. Figure 1: Reactivity of RhAl 2 O 4–6 + clusters with CO. Time-of-flight mass spectra for reactions of mass selected RhAl 2 O 4–6 + with N 2 ( a , e , g ) and CO ( b – d , f , h ) are shown. Peaks marked with asterisk and hollow circle in d are CO adsorption products of RhAl 2 OCO + and RhAl 2 O 2 CO + , respectively. Rh x Al y O z + and Rh x Al y O z X + ( X =N 2 , CO and H 2 O) species are labeled as x,y,z and x,y,zX , respectively. Signal 1,2,4H 2 O in h is due to the residual water in the gas handling system. The time periods for reactions RhAl 2 O 6 + + CO, RhAl 2 O 5 + + CO and RhAl 2 O 4 + + CO were about 1.1, 0.7 and 0.6 ms, respectively. The reactant gas pressures are shown in mPa. 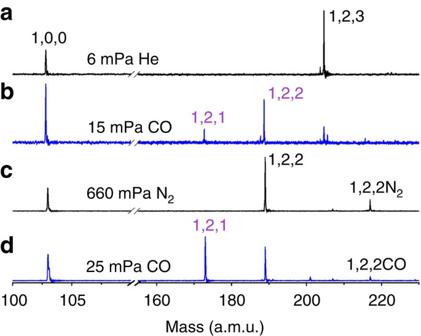Figure 2: Reactivity of RhAl2O2–3+clusters with CO. Time-of-flight mass spectra for reactions of mass selected RhAl2O2–3+with He (a), N2(c) and CO (b,d) are shown. The time period was∼0.6 ms for both reactions. Full size image Figure 2: Reactivity of RhAl 2 O 2–3 + clusters with CO. Time-of-flight mass spectra for reactions of mass selected RhAl 2 O 2–3 + with He ( a ), N 2 ( c ) and CO ( b , d ) are shown. The time period was ∼ 0.6 ms for both reactions. Full size image The strong signals that can be assigned as RhAl 2 O 4 CO + and RhAl 2 O 4 (CO) 2 + ( Fig. 1a–d ) on the interaction of RhAl 2 O 6 + with CO indicate the displacement of the O–O unit in RhAl 2 O 6 + by CO, which is more facile than N 2 displacement ( Fig. 1a ), and further demonstrates the presence of O 2 −· or O 2 2− unit in RhAl 2 O 6 + . Each of the cluster source generated RhAl 2 O m + ( m =5−2) clusters could also react with CO to generate products, from RhAl 2 O m −1 + to RhAl 2 O + ( Figs 1f,h and 2b,d ). This provides convincing evidence that RhAl 2 O 6 + can indeed oxidize five CO molecules consecutively. The pseudo-first-order rate constants ( k 1 , in unit of 10 −10 cm 3 per molecule per second) on the interaction of RhAl 2 O m + ( m =6–2) cluster ions with CO can be well fitted ( Fig. 3 ) and the determined rate constants are presented in Supplementary Table 1 . The rate constants for the reactions of the cluster source generated RhAl 2 O m + ( m =6–2) with CO are 4.9±1.5 ( m =6), 6.2±1.9 ( m =5), 1.6±0.5 ( m =4), 6.9±2.0 ( m =3) and 2.4±0.7 ( m =2), which correspond to the reaction efficiencies [30] of about (37±11)%, (47±14)%, (13±4)%, (54±16)% and (19±6)%, respectively. Furthermore, we note that the clusters with odd number of oxygen atoms such as RhAl 2 O 5 + are more reactive towards CO oxidation than clusters with even number of oxygen atoms such as RhAl 2 O 6 + . 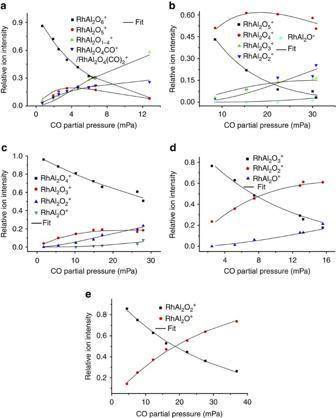Figure 3: Reaction kinetics. Variation of ion intensities with respect to the partial pressures of CO in RhAl2Om+(m=6−2) + CO are shown (a–e). The solid lines are fitted to the experimental data points by the least-square procedure. The Rh+(1,0,0) ions (Fig. 2) are mostly generated during cooling of the RhAl2O3+and RhAl2O2+cluster ions through collisions with He gas in the ion trap reactor; thus, the ion intensity of Rh+(nearly independent on the CO partial pressure) is excluded in the fitting. SeeSupplementary Table 1for details of the determined rate constant values. Figure 3: Reaction kinetics. Variation of ion intensities with respect to the partial pressures of CO in RhAl 2 O m + ( m =6−2) + CO are shown ( a – e ). The solid lines are fitted to the experimental data points by the least-square procedure. The Rh + (1,0,0) ions ( Fig. 2 ) are mostly generated during cooling of the RhAl 2 O 3 + and RhAl 2 O 2 + cluster ions through collisions with He gas in the ion trap reactor; thus, the ion intensity of Rh + (nearly independent on the CO partial pressure) is excluded in the fitting. See Supplementary Table 1 for details of the determined rate constant values. Full size image Reaction mechanism The density functional theory calculated thermodynamic data for CO oxidation by RhAl 2 O m + ( m =2–6) are shown in Fig. 4 . The overall oxidation (RhAl 2 O 6 + + 5CO → RhAl 2 O + + 5CO 2 ) is highly exothermic (−9.00 eV). The low-lying energy isomers of clusters RhAl 2 O m + ( m =6–1) are provided in Supplementary Figs 1–6 . The lowest energy isomer of RhAl 2 O 6 + is in the triplet spin state ( Supplementary Fig. 1 ) and contains a superoxide O 2 −· unit (O–O bond: 137 pm; Fig. 5 ). The existence of O 2 −· unit in RhAl 2 O 6 + is consistent with the appearance of RhAl 2 O 4 N 2 + and RhAl 2 O 4 CO + (or RhAl 2 O 4 (CO) 2 + ) on the interaction of RhAl 2 O 6 + with N 2 and CO ( Fig. 1a–d ), respectively. Supplementary Figs 7 and 8 show that the Al-site adsorption contributes to the displacement of the O 2 −· unit in RhAl 2 O 6 + by N 2 or CO and both reactions are calculated to be thermodynamically and kinetically favourable, and CO displacement is more facile than N 2 displacement. This is consistent with the relatively higher intensity of RhAl 2 O 4 CO + (or RhAl 2 O 4 (CO) 2 + ) than RhAl 2 O 4 N 2 + observed in the experiment ( Fig. 1a–d ). The positively charged Rh in RhAl 2 O 6 + (natural charge: +1.14 e ) can trap CO tightly at the first step (I1, Δ H 0 =−1.49 eV; Fig. 5 ) and then the oxidation of CO (I1→TS1→I2) by the highly reactive atomic oxygen radical anion O −· (ref. 31 ) takes place. Direct CO oxidation by the O 2 −· unit has to suffer from a positive barrier of 0.03 eV, which is much less favourable than the oxidation by O −· . The Rh atom in product RhAl 2 O 5 + (denoted as P RhAl 2 O 5 + , the structure of which is different from the lowest energy structure; Supplementary Fig. 2 ) can capture another CO tightly (I3, binding energy of −2.18 eV). Formation of the bent CO 2 is the bottleneck (I3→TS2→I4) for CO oxidation by P RhAl 2 O 5 + . This step is to subject to a barrier of 1.26 eV. The subsequent steps follow a nearly downhill pathway characterized by small barriers to yield RhAl 2 O 4 + and CO 2 ( Supplementary Fig. 9 ). Furthermore, theoretical calculations show that the energy of the critical transition state for reaction RhAl 2 O 5 + + CO (−0.47 eV; Supplementary Fig. 10 ) is lower with respect to that for reaction RhAl 2 O 6 + + CO (TS1, −0.37 eV; Fig. 5 ). This can well interpret the more reactive behaviour of the cluster source-generated RhAl 2 O 5 + than RhAl 2 O 6 + in the experiment. 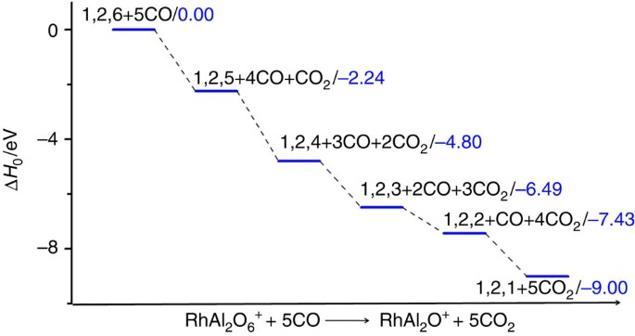Figure 4: Reaction thermodynamics. Density functional theory (DFT)-calculated thermodynamic data for CO oxidation by RhAl2O2–6+. The energies are zero-point vibration-corrected in unit of eV. Figure 4: Reaction thermodynamics. Density functional theory (DFT)-calculated thermodynamic data for CO oxidation by RhAl 2 O 2–6 + . The energies are zero-point vibration-corrected in unit of eV. 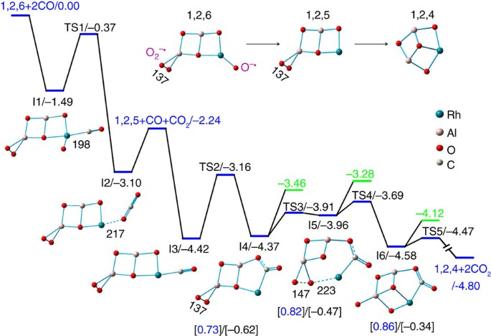Figure 5: Structures and reaction mechanisms. Density functional theory (DFT)-calculated potential energy profiles for the oxidation of the first two CO molecules by RhAl2O6+. The lowest energy structure of RhAl2O6+(1,2,6) and the productsPRhAl2O5+(1,2,5) and RhAl2O4+(1,2,4) are provided. Symbols O2−·and O−·denote superoxide and atomic oxygen radical species, respectively. The relative energies for intermediates (I1–I6) and transition states (TS1–TS5) are in unit of eV. Structures of I1–I6 are shown. Bond lengths are given in pm. The values in green show the relative energies for direct CO2desorption from I4 to I6. The values in the square brackets show the natural charges on Rh (blue) and CO2unit (black). See alsoSupplementary Figs 9–13for more information. Full size image Figure 5: Structures and reaction mechanisms. Density functional theory (DFT)-calculated potential energy profiles for the oxidation of the first two CO molecules by RhAl 2 O 6 + . The lowest energy structure of RhAl 2 O 6 + (1,2,6) and the products P RhAl 2 O 5 + (1,2,5) and RhAl 2 O 4 + (1,2,4) are provided. Symbols O 2 −· and O −· denote superoxide and atomic oxygen radical species, respectively. The relative energies for intermediates (I1–I6) and transition states (TS1–TS5) are in unit of eV. Structures of I1–I6 are shown. Bond lengths are given in pm. The values in green show the relative energies for direct CO 2 desorption from I4 to I6. The values in the square brackets show the natural charges on Rh (blue) and CO 2 unit (black). See also Supplementary Figs 9–13 for more information. Full size image The key step for the transfer of five oxygen atoms from RhAl 2 O 6 + to CO lies in the facile dissociation of the O 2 −· unit in P RhAl 2 O 5 + . Dissociation of the chemically adsorbed molecular O 2 (superoxide O 2 −· or peroxide O 2 2− ) is often considered to be the crucial step in oxidation reactions [32] . Recent gas-phase studies indicated that a single Au atom in AuTi 3 O 8 −22 is not enough to promote the dissociation of the O 2 2− unit, while the Au dimer in Au 2 VO 4 − can promote O 2 2− unit dissociation or direct participation in CO oxidation [25] . In this study, a single Rh atom in P RhAl 2 O 5 + can promote the dissociation of the O 2 −· unit and the process is much more favourable than CO 2 desorption ( Fig. 5 ). This is rationalized by the strong Rh–C multiple bonds (5.97 eV) [33] and the strong Rh–O bond (4.16 eV) [34] . Thus, the Al–O 2 −· unit in I4 can approach the Rh atom favourably to form structure Al–O 2 2− ˙˙˙Rh–CO 2 in I5. The elongation of the O–O bond from 137 pm in I4 to 147 pm in I5 is a good indicator for the activation of the superoxide O 2 −· to peroxide O 2 2− unit. The structure of I5 is crucial to induce further electron flowing into the O 2 2− unit from both of the Rh atom and the CO 2 unit ( Fig. 5 ), and then the O 2 2− unit can be dissociated favourably to produce O 2− –Al–O 2− –Rh–CO 2 (I5→TS4→I6). Direct oxidation of CO by the O 2 −· unit in P RhAl 2 O 5 + ( Supplementary Fig. 9 ) is less favourable than the pathway in Fig. 5 . This is consistent with previous study that instead of the direct participation in CO oxidation, molecular oxygen adsorbs at the interface between the oxygen vacancy and the single Rh site and then is followed by facile dissociation [35] . Release of three additional oxygen atoms from the resulting RhAl 2 O 4 + to CO are calculated to be thermodynamically and kinetically favourable ( Supplementary Figs 11–13 ). In each of these OAT steps, Rh atom functions as the preferred trapping site to anchor CO and then delivers CO for oxidation by the oxygen atoms in direct connection with Rh. The theoretical calculations well interpret the unique reactivity of RhAl 2 O 6 + observed in the experiment. Metal-mediated OAT reaction is usually accompanied with the reduction of central metal by electrons that are stored originally in the removed oxygen atoms [36] (equation (2)). The positively charged metal centre is crucial to provide not only the characteristic site for the adsorption of CO (ref. 37 ) but also the oxidative centre to accept electrons. Recent gas-phase studies highlighted that the cleavage of Au–O bond and the formation of Au– M bond ( M =Al, V, Ti, and Fe) is of great importance in CO oxidation by Au-doped clusters [22] , [23] , [24] , [25] . However, each of the Au-doped clusters can oxidize only one or at most two CO molecules and then the polarity conversion of Au atom from positive to negative takes place because of the formation of the reductive Au– M bond. In sharp contrast, natural charge analysis demonstrates that after the transfer of four oxygen atoms from RhAl 2 O 6 + to CO, the Rh atom is still positively charged (+0.53 e , Fig. 6 ) in product RhAl 2 O 2 + , which can also oxidize a CO molecule. The natural charge on Rh atom is decreased from +1.14 e in RhAl 2 O 6 + to +1.00 e in P RhAl 2 O 5 + after the oxidation of the first CO. In this step, Rh acts as the primary centre to accumulate the electron that is localized originally on O −· radical, as shown from the change of spin density distribution, RhAl 2 O 6 + versus P RhAl 2 O 5 + . However, the Rh atom is re-oxidized in product RhAl 2 O 4 + (+1.15 e ) after the oxidation of the second CO due to the dissociation of the O 2 −· unit (I4→I5→I6; Fig. 5 ). This step is crucial to recover the oxidative reactivity of Rh. In situ Raman spectroscopic study also demonstrated that supported Rh oxide can oxidize CO and then the Rh oxide is subsequently re-oxidized by the oxygen atoms from oxide support [7] . This phenomenon can be traced back to the well-fitting strength of Rh–O bond (4.16 eV) [34] , which is strong enough to promote the dissociation of the O 2 −· unit in P RhAl 2 O 5 + and prevent the formation of the reductive Rh–Al bond (3.26 eV, by theoretical calculation) in RhAl 2 O 2–6 + but at the same time is relatively weak to deliver oxygen atoms to oxidize CO (O–CO: 5.52 eV) [38] . Previous studies show that Rh prefers to coordinate not only with the surface oxygen atoms but also the subsurface oxygen in oxide support [35] . The strong Rh–O bond inhibits the migration of Rh atom to the oxygen vacancy and remains positively charged. Using high-resolution in situ X-ray diffraction and transmission electron microscopy, Stierle and colleagues [1] reported the reversible and oxygen-induced shape transformation of Rh nanoparticles by the formation of O–Rh–O surface oxide during the cycle of catalytic CO oxidation. In contrast, the stronger Au–M (Au–Al=3.37 eV (ref. 39 ), Au–V=2.49 eV (ref. 38 ) and Au–Ti=2.56 eV (by theoretical calculation)) than Au–O bond (2.27 eV) [34] facilitates the formation of the reductive Au–M bond after the oxidation of only one or two CO molecules. 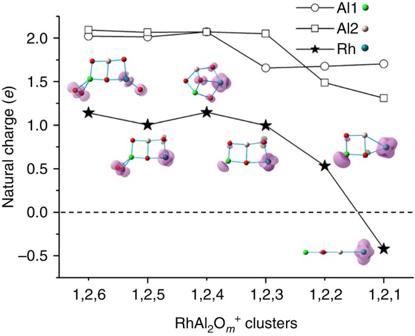Figure 6: Natural charge. Density functional theory (DFT)-calculated natural charges (e) on the Rh atom and Al atoms in RhAl2O1–6+. The spin density distributions on individual atoms are shown in the purple isosurfaces. Figure 6: Natural charge. Density functional theory (DFT)-calculated natural charges ( e ) on the Rh atom and Al atoms in RhAl 2 O 1–6 + . The spin density distributions on individual atoms are shown in the purple isosurfaces. Full size image The negatively charged Rh has been theoretically predicted [40] and experimentally postulated [41] . The RhAl 2 O + cluster is a linear structure (Al–O–Al–Rh) and the single oxygen atom is sandwiched between two Al atoms. This structure with triplet spin state has been confirmed to be the lowest energy isomer of RhAl 2 O + by more accurate CCSD(T) calculation ( Supplementary Fig. 6 ). The two unpaired electrons are mainly localized on the Rh atom ( ∼ 1.83 μ B , Fig. 6 ), indicating that such Rh atom can be considered to be Rh −1 (4 d 9 5 s 1 ). The electron configuration calculations (4 d 8.75 5 s 0.64 5 p 0.03 ) provide solid evidence for the negatively charged Rh in RhAl 2 O + . Thus, the oxidation state of Rh changes from +2.5 in RhAl 2 O 6 + to −1 in RhAl 2 O + (calculated based on the distribution of spin density; Fig. 6 ) during the transfer of five oxygen atoms from RhAl 2 O 6 + to CO. This rather large range of Rh oxidation state changes in chemical reactions has rarely been reported (the Au oxidation state changes from +1 to −1), covering from cationic to anionic, and it is the driving force to accumulate the electrons that are stored originally in the released oxygen atoms and promotes the unique oxidative reactions to proceed. In conclusion, we have demonstrated that a single atom of Rh can unexpectedly promote the transfer of five oxygen atoms to oxidize CO from a nine-atom cluster RhAl 2 O 6 + . This study leads a leap ahead towards OAT reactions in the field of cluster science and represents an important step to understand the participation of lattice oxygen promoted by noble metals. The preferable Rh–O rather than the reductive Rh–Al bond formation together with the capability of Rh to accumulate the large amounts of electrons are crucial factors to drive the unique reactions. This gas-phase study reveals the molecular-level origin for the puzzling experimental observation that trace amounts of Rh can promote the reactivity of lattice oxygen of Al 2 O 3 (refs 4 , 5 , 9 ), a chemically very inert material. Cluster generation and reactivity detection The Rh x Al y O z + cluster ions were generated by laser ablation of a mixed-metal disk compressed with Rh and Al powders (molar radio Rh/Al=1/1) in the presence of O 2 (0.4%) seeded in a He carrier gas with a backing pressure of 6.0 standard atmospheres. The cluster ions of interest were mass selected using a quadrupole mass filter and then entered into a linear ion trap (LIT) reactor, where they were cooled by collisions with a pulse of He gas and then interacted with a pulse of 5% (for reactions RhAl 2 O m + ( m =2–5) + CO) or 2% (for reaction RhAl 2 O 6 + + CO) CO seeded in He for around 0.6 ∼ 1.1 ms. The temperature of cooling gas (He), reactant gases (CO or N 2 ) and the LIT reactor was around 298 K. The cluster ions ejected from the LIT were detected by a reflector time-of-flight mass spectrometer. The details of running the time-of-flight mass spectrometer [42] , quadrupole mass filter [43] and the LIT [44] can be found in our previous works. Rate constant fitting Equation (3) was used to determine the pseudo-first-order rate constants ( k 1 ) of cluster reactions in an ion trap reactor [44] , in which I R is the signal intensity of the reactant cluster ions, I T is the total ion intensity including product ion contribution, k B is the Boltzmann constant, T is the temperature ( ∼ 298 K), t R is the reaction time and P is the effective pressure of the reactant gas in the ion trap reactor. To calculate the reaction efficiencies (the possibilities of reaction on each collision), the collision rate constants were calculated on the basis of the surface charge capture model developed in the literature [30] . It is noteworthy that for reaction RhAl 2 O 5 + + CO, the relative ion intensity of RhAl 2 O 5 + is the reactive component generated in the experiment and the unreactive component is not included. The unreactive component of RhAl 2 O 5 + could be well-fitted by equation (4) [45] . in which x inert is the relative intensity of the unreactive component of RhAl 2 O 5 + and k 1 is the pseudo-first-order rate constant of the reactive component of RhAl 2 O 5 + . The x inert was determined to be about 12%, indicating that the experimentally generated RhAl 2 O 5 + may have isomers that are not or less reactive with CO. Computational details Density functional theory calculations using the Gaussian 09 (ref. 46 ) programme were carried out to investigate the mechanistic details on the oxidation of five CO molecules by a nine-atom rhodium–aluminum oxide cluster (RhAl 2 O 6 + ). To find an appropriate functional for the Rh–Al–O system, the bond dissociation energies of Rh–O, Rh–C, Al–O, O–O, Rh–Al and O–CO were computed by various functionals and compared with available experimental data ( Supplementary Table 2 ). It turns out that M06L [47] was the best overall; thus, the results by M06L were given throughout the work. The TZVP basis set [48] for Al, C and O atoms and a D95V basis set [49] combined with the Stuttgart/Dresden relativistic effective core potential (denoted as SDD in Gaussian software) for Rh atom were used in all the calculations. A Fortran code based on a genetic algorithm [50] was used to generate initial guess structures of RhAl 2 O 1–6 + . The reaction mechanisms were studied for RhAl 2 O 6 + + 5CO → RhAl 2 O + + 5CO 2 . The relaxed potential energy surface scan was used extensively to obtain good guess structures for intermediates and transition states along the pathways. The transition states were optimized using the Berny algorithm [51] . Intrinsic reaction coordinate calculations [52] , [53] were performed so that each transition state connects two appropriate local minima. Vibrational frequency calculations were carried out to check that intermediates and transition state have zero and only one imaginary frequency, respectively. How to cite this article: Li, X.-N. et al . A nine-atom rhodium–aluminum oxide cluster oxidizes five carbon monoxide molecules. Nat. Commun. 7:11404 doi: 10.1038/ncomms11404 (2016).